Direct observation of dual-step twinning nucleation in hexagonal close-packed crystals 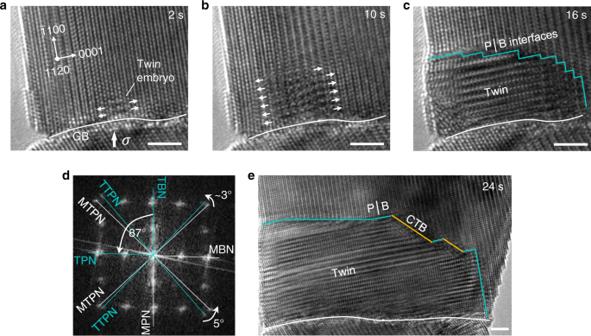Fig. 1: Direct observation of a twinning nucleation process. a–cSequential HRTEM images showing twinning nucleation in a HCP rhenium nanocrystal under < 1 −1 0 0 > -oriented compression. Arrows indicate the expansion of basal layers in the twin embryo. Turquoise lines indicate the Prismatic│Basal (P│B) interfaces between the twin embryo and matrix. White lines indicate the grain boundary (GB). Block arrow inaindicates the loading direction.dFast Fourier transformation of the twin embryo inc. TBN, MPN, TPN, MBN, TTPN, and MTPN mean the plane normal directions of twin basal, matrix prismatic, twin prismatic, matrix basal, twin twinning plane and matrix twinning plane, respectively.eMorphology of the twin as it grew. Yellow lines indicate the coherent twin boundaries (CTB). Scale bars ina–c,e, 2 nm. Design and processing of advanced lightweight structural alloys based on magnesium and titanium rely critically on a control over twinning that remains elusive to date and is dependent on an explicit understanding on the twinning nucleation mechanism in hexagonal close-packed (HCP) crystals. Here, by using in-situ high resolution transmission electron microscopy, we directly show a dual-step twinning nucleation mechanism in HCP rhenium nanocrystals. We find that nucleation of the predominant {1 0 −1 2} twinning is initiated by disconnections on the Prismatic│Basal interfaces which establish the lattice correspondence of the twin with a minor deviation from the ideal orientation. Subsequently, the minor deviation is corrected by the formation of coherent twin boundaries through rearrangement of the disconnections on the Prismatic│Basal interface; thereafter, the coherent twin boundaries propagate by twinning dislocations. The findings provide high-resolution direct evidence of the twinning nucleation mechanism in HCP crystals. Twinning, on par with dislocation, is an essential carrier of crystal deformation [1] , [2] . Particularly, in hexagonal close-packed crystals (e.g., magnesium, titanium, and rhenium), it is required to mediate deformation along the < c > axis of the crystal structure [3] , [4] , [5] . By creating coherent twin boundaries (CTB) within a crystal, twinning can significantly affect the physical properties of the crystal. For instances, twin architectures can confine dislocation activities and effectively increase the strength of metals without sacrificing their ductility [6] , [7] , [8] , [9] . As such, the atomic mechanism of twinning nucleation—the key to control twinning—has drawn extensive research interest [4] , [10] , [11] , [12] , [13] , [14] , [15] , [16] . Unfortunately, owing to a lack of direct experimental evidence, current knowledge on twinning nucleation in HCP crystals remains at the level of debatable theories. Given that the reliability of simulations and topological analysis critically depends on a correct description of interatomic potentials [17] , [18] , and that ex situ static characterization may be misleading owing to the high tendency of detwinning upon unloading [19] , [20] , it is generally believed that in situ atomic scale investigations are indispensable for unraveling the mystery of twinning nucleation. As more than one atom exists in the motif of the HCP crystal, shear alone cannot move all atoms to their correct positions in the twin; additional atomic adjustments (called shuffles) are always required in the twinning process [17] , which not only significantly affects the dynamic process of twinning [13] , [18] , [21] , [22] but also poses tremendous challenges on direct atomic interrogation. Here, by using advanced crystal manipulation techniques and in situ high-resolution transmission electron microscopy (HRTEM), twinning nucleation processes in HCP rhenium nanocrystals are directly captured at atomic resolution. It is revealed that the {1 0 −1 2} <1 0 −1 −1> twinning nucleates through a dual-step mechanism lead by transformations of parent prismatic (P) planes into the twin basal (B) planes; this process establishes the lattice correspondences of the twin plus a minor rotational deviation from the ideal parent–twin mutual-orientation; subsequently, ideal twin forms by the rearrangement of interfacial defects on the P│B interfaces and ensuing formation of CTB. The findings provide direct evidences to the twinning nucleation mechanism in HCP crystals. Prismatic-to-basal transformation Fig. 1a (and Supplementary Movie 1 ) shows a {1 0 −1 2} twinning nucleation process from the grain boundary of a rhenium (Re) bi-crystal under compression. Incipient plastic deformation started with the nucleation of a {1 0 −1 2} twin embryo at a local region of the grain boundary (where stress concentration might be present). The twin embryo was ~1 nm in dimension upon nucleation, i.e., containing only a few unit-cells, and grew by formation and lateral expansion of new basal layers on the twin/matrix interface (Fig. 1a–c ). As it grew through the sample thickness direction, atomic-resolution image of the twin embryo was captured (see Fig. 1c ), demonstrating that the laterally expanding layers were indeed basal planes. During this process, the {1 0 −1 2} twinning planes in the parent and twin crystals were not parallel (Fig. 1d ), implying that the observed process in Fig. 1a–c was not dominated by twinning dislocations [1] , [23] . As the twin embryo grew in subsequent compression, CTB on the {1 0 −1 2} plane were formed (Fig. 1e ), demonstrating that the prior transformation was indeed an incipient stage of the twinning nucleation. Same mechanism of twinning nucleation was also identified frequently on the side surfaces of different samples (see Supplementary Fig. 1 ). Fig. 1: Direct observation of a twinning nucleation process. a – c Sequential HRTEM images showing twinning nucleation in a HCP rhenium nanocrystal under < 1 −1 0 0 > -oriented compression. Arrows indicate the expansion of basal layers in the twin embryo. Turquoise lines indicate the Prismatic│Basal (P│B) interfaces between the twin embryo and matrix. White lines indicate the grain boundary (GB). Block arrow in a indicates the loading direction. d Fast Fourier transformation of the twin embryo in c . TBN, MPN, TPN, MBN, TTPN, and MTPN mean the plane normal directions of twin basal, matrix prismatic, twin prismatic, matrix basal, twin twinning plane and matrix twinning plane, respectively. e Morphology of the twin as it grew. Yellow lines indicate the coherent twin boundaries (CTB). Scale bars in a – c , e , 2 nm. Full size image Zoom-in view of another {1 0 −1 2} twinning nucleation process demonstrates that expansion of the twin basal layers is actually mediated by disconnections on the P│B interfaces [24] (Fig. 2a–d ). Most of these disconnections showed a step height of two atomic layers (Fig. 2b–c ); during their migration, the parent prismatic planes transformed into twin basal planes (P → B transformation) following a one-to-one planar correspondence (as evidenced by the atomic-resolution images in Fig. 2e–f ). Fig. 2: Twin embryo growth mediated by disconnections on the P│B interfaces. a – d Sequential HRTEM images showing the process. The zig-zag turquoise lines indicate the P│B interfaces, wherein the step features are disconnections on the P│B interface. Arrows indicate the moving direction of the disconnections. e Atomic-resolution HAADF-STEM image of the P│B-type twin boundaries and f corresponding inverse fast Fourier transformation showing one-to-one correspondence between twin basal planes and matrix prismatic planes. Insets in e ) show the atomic models of the two types of plane. The zig-zag turquoise lines in e , f indicate the P│B interfaces. Scale bars in a – d , 1 nm; scale bars in e – f , 2 nm. Full size image The deviation from an ideal {1 0 −1 2} twin Though the P → B transformation does not establish ideal parent–twin mutual-orientation (Fig. 1d ), it establishes exactly the same lattice correspondence as that of an ideal {1 0 −1 2} twin [25] (as schematically depicted by unit-cell level analysis in Fig. 3 ). To track the lattice correspondences, the prismatic plane, basal plane, twinning plane, and conjugate twinning plane are color-coded (Fig. 3a–b ). In the observed mechanism, the parent P plane transforms into twin B plane, and the parent B plane transforms into twin P plane (Fig. 3c ). As such, the twinning plane is rotated by ~4 o during the transformation. By contrast, position of the twinning plane is invariant in the ideal {1 0 −1 2} twinning (Fig. 3d ). Clearly, the lattice correspondences generated by the two mechanisms are exactly the same (Fig. 3e–f ), except for a minor rotation depending on the magnitude of twinning shear (Supplementary Fig. 2 ). In other words, the P → B transformation completes the twinning process in the sense that it moves all atoms in parent structure to their correct positions in the twin. Fig. 3: Schematic illustration of the dual-step twinning nucleation mechanism. a Unit-cell of a HCP structure. Solid balls represent individual atoms. b <1 1 −2 0 > -projection view of the unit-cell. The prismatic plane (P), basal plane (B), twinning plane (K 1 ), and conjugate twinning plane (K 2 ) are colored magenta, blue, yellow, and turquoise, respectively, for easy tracking of their corresponding planes after the transformations. Arrows in c , d indicate the atomic movements required to accomplish the transformations of the unit-cell; in particular, blue arrows in d indicate the portion that delivers the homogeneous shear. e Twin embryo structure generated by the P → B transformation, which shows a minor rotational deviation compared with the ideal twin f . Angle of the minor rotation can be described by tan −1 ( s /2), where s is the magnitude of twinning shear (see Supplementary Fig. 2 for the derivation). Full size image Correction of the deviation Interestingly, the minor rotational deviation from the ideal twin–parent mutual-orientation can be corrected by subsequent transformations. As shown in Fig. 4a–c , the disconnections on the P│B interfaces rearranged to align on the twinning plane upon unloading, forming CTB. Same transformation of twin boundaries can also happen during the twin embryo growth (Fig. 1e ). This is essentially a twin boundary faceting process driven by twin boundary energy minimization [14] , [24] , [26] , [27] . More importantly, the orientation relation between the twin and matrix became ideal at very local regions thereafter (see Supplementary Fig. 3 ). Subsequent movement of the CTB was mediated by conventional ( b 2 , h 2 ) twinning dislocations (see Fig. 4d–g for that in a detwinning process and Supplementary Fig. 4 for that in a twinning process), manifesting a long-desired direct evidence to the classical mechanism of {1 0 −1 2} twinning [14] , [22] , [28] . Fig. 4: Twin boundary transformation from P│B interfaces to CTB during detwinning. a – c Sequential HRTEM snapshots of the process. The dominant defects in the twinning transit from disconnections on P│B interfaces to twinning dislocations ( b 2 , h 2 ) on CTB. Zig-zag turquoise lines indicate the P│B interfaces. White arrows in a , b indicate the moving directions of the disconnections on the P│B interface. d Overview of the twin upon partial detwinning, showing serrated twin boundaries. e – g Sequential HRTEM snapshots showing CTB propagation by twinning dislocations. White dash line is a reference line to show the migration of the CTBs (colored lines). Arrows in c , e – g indicate the migration direction of the twinning dislocations. Scale bars in a – g , 2 nm. Full size image The dual-step mechanism of twinning nucleation In retrospect, above observations directly demonstrate a dual-step mechanism of the {1 0 −1 2} twinning nucleation: (I) establishment of the lattice correspondence through P → B transformation, and then (II) correction of the minor rotational deviation through twin boundaries transformation. Note that the formation process of the incipient unit-cell-scale twin embryo (Fig. 1a ) is shrouded by the parent lattice along the TEM electron beam direction; based on the observation that it is a P → B transformation process, the unit-cell-scale embryo is likely formed by the pure-shuffle mechanism [11] , [14] . It should be noted that the side surface of the nanocrystal can facilitate the P → B transformation by providing accommodation for the lateral deformation especially when the transformation propagates to the side surface. This is evidenced by the bulge on the left-side surface in Fig. 1c and the fact that P → B transformation played a major role in mediating the {1 0 −1 2} twinning nucleation and growth in our nanosized samples and CTB is only occasionally formed during the process. In the confined environment of bulk samples, accommodation mechanisms other than the side surface are needed to facilitate the P → B transformation, such as elastic and plastic deformation in front of the twin boundary [29] , deformation of the neighboring grains [30] , intersection region of the grain boundaries [31] and formation of threading dislocations on the P│B interface [27] , [32] . Considering the fact that the incipient nucleation is a local event at atomic scale, one or more of these mechanisms should be able to accommodate the limited deformation, resulting from the initial P → B transformation as a leading step of twinning nucleation. This is supported by the fact that initial nucleus of the twin in our experiment is away from (and without obviously bulging) the side surface (Fig. 1a–b ). Above all, the dual-step manner of the twinning nucleation should persist in the interior of the bulk samples. Though, the energy barrier for the same mechanism happening close to the free surface or in the bulk of the aggregate should be different. Compared with the free side surface, the above strain accommodation mechanisms in bulk samples likely requires a higher stress to be active; therefore, growth of the twin nucleus by continuous P → B transformation may be limited and the classical shear of twinning dislocations on the CTB may become prevalent in bulk samples. In addition, our observation does not disprove other twinning nucleation models (e.g., reaction and dissociation of matrix dislocations [33] , [34] , [35] , [36] , surface/interface emission of twinning dislocations [10] , [30] , [37] , [38] ); the nanoscale dimension of the crystals here prompts the starvation of matrix dislocations [39] , [40] , [41] , eliminating potential twinning nucleation through the pole-mechanism [33] , [34] , or dislocation dissociation [35] , [36] . It may also inhibit the nucleation of twinning dislocations from the side surface [41] . Moreover, the bi-nanocrystal sample geometry has much less grain boundaries than a bulk polycrystalline sample and may significantly reduce the availability of favorable nucleation sites for twinning dislocations [10] , [42] . Though our finding is based on Re nanocrystals, it can be reasonably extended to other bulk HCP metals. First, the observations provide a direct understanding on the origin of the serrated twin boundaries in many bulk HCP metals including Co [21] , [43] , [44] , [45] , [46] , Ti [47] , [48] , Mg [32] , [49] , [50] , Zn [29] , [51] , [52] . Second, it is well known that c/a ratio has critical influence on the deformation of HCP metals [5] ; as the c/a ratio of Re (1.615) is very close to those of Mg (1.624) and Ti (1.588), it is reasonable to expect the observed twinning nucleation mechanism in these metals (see Supplementary Fig. 2 for further discussion). Third, the dual-step twinning nucleation mechanism offers another fundamental understanding to the fact that the active twinning variant in HCP metals is not always associated with the largest resolved shear stress on the twinning plane [18] , [42] , [53] . As the onset of P → B transformation depends on the normal stresses on the prismatic/basal planes which, in most cases, translate to both a resolved shear stress and a normal stress on the twinning plane, twinning nucleation by the dual-step mechanism can also be critically affected by the normal stress on the twinning plane. Finally, a major advantage of nanoscale samples over bulk sample is that high-stress states can be attained [54] ; localized stress concentrations within bulk samples may provide equivalent stress condition for the activation of the dual-step mechanism. Moreover, our findings provide a solid fundamental basis for the twinning-based design and processing of advanced HCP alloys. Since the {1 0 −1 2} twinning starts at low stress-state and has crucial role in the early stage deformation of magnesium alloys [18] , [55] , it is critical to impede the easy nucleation or growth of {1 0 −1 2} twins for strengthening the magnesium alloys. Based on the findings here, an effective way to do this is through cyclic deform-unload-anneal processing. 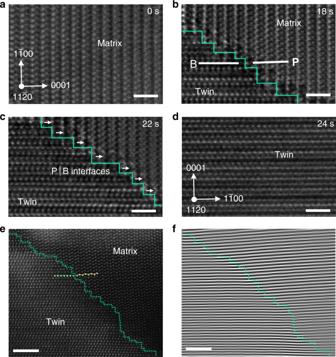Fig. 2: Twin embryo growth mediated by disconnections on the P│B interfaces. a–dSequential HRTEM images showing the process. The zig-zag turquoise lines indicate the P│B interfaces, wherein the step features are disconnections on the P│B interface. Arrows indicate the moving direction of the disconnections.eAtomic-resolution HAADF-STEM image of the P│B-type twin boundaries andfcorresponding inverse fast Fourier transformation showing one-to-one correspondence between twin basal planes and matrix prismatic planes. Insets ine) show the atomic models of the two types of plane. The zig-zag turquoise lines ine,findicate the P│B interfaces. Scale bars ina–d, 1 nm; scale bars ine–f, 2 nm. In the deform-unload process, {1 0 −1 2} twins nucleates and propagate; upon unloading, the twin boundaries retreat and relocate to the CTB (as demonstrated in Fig. 4 and Supplementary Fig. 3 ). In the subsequent anneal process, the alloying elements will gradually segregate on the CTB [6] and pin these boundaries from further propagation. Then, the future deformation would require nucleation of new {1 0 −1 2} twins rather than propagation of existing {1 0 −1 2} twins. As such, the easy nucleation sites for {1 0 −1 2} twinning can be gradually depleted by cyclic deform-unload-anneal processing. Increasing the interfacial energy of P│B-type interfaces [27] (e.g., by alloying) raises the formation energy of the twin embryo and hence makes it harder for the {1 0 −1 2} twinning nucleation through the observed mechanism. Moreover, hierarchical twin structures may be enabled by patterning desired defects for twinning nucleation. Per Fig. 3c , the P → B transformation correlates to a compressive strain on the prismatic plane, suggesting that normal strain fields from the defects may be used to control the twinning nucleation. Consistently, we captured a twinning nucleation event at the compressive strain field of a dislocation core (Fig. 5 and Supplementary Fig. 5 ). As revealed by quantitative geometrical phase analysis [56] (Fig. 5e ), the dislocation in Fig. 5a generated compressive strains on the prismatic planes to the right of the dislocation core; in the subsequent compression of the crystal, a {1 0 −1 2} twinning preferentially nucleated at the region where compressive strain of the dislocation core was the largest, demonstrating that the strain field of matrix dislocations could prompt the twinning nucleation. It should be noted that a high compressive stress (~5 GPa based on a rough estimation [57] ) was attained at the moment of the twinning nucleation in Fig. 5b , which is not readily available in polycrystalline Re samples without significant stress concentrations [30] . Though, similar mechanism is expected to be present in nano-grains of HCP metals wherein high-stress-state can be attained. Fig. 5: Twinning nucleation assisted by the strain field of a matrix dislocation. a – d Sequential HRTEM images showing the nucleation of a twin embryo near the dislocation core (indicated by the “├” symbol). The crystal was under <1 −1 0 0 > -oriented compression and viewed along the <1 1 −2 0> direction. White dashed line in a is the Burgers circuit which indicates an < a > component in the Burgers vector (indicated by the yellow arrow) of the dislocation. Detailed analysis of the Burgers vector is shown in Supplementary Fig. 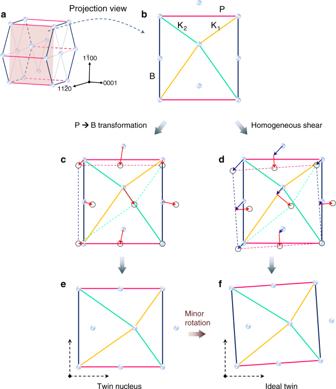Fig. 3: Schematic illustration of the dual-step twinning nucleation mechanism. aUnit-cell of a HCP structure. Solid balls represent individual atoms.b<1 1 −2 0 > -projection view of the unit-cell. The prismatic plane (P), basal plane (B), twinning plane (K1), and conjugate twinning plane (K2) are colored magenta, blue, yellow, and turquoise, respectively, for easy tracking of their corresponding planes after the transformations. Arrows inc,dindicate the atomic movements required to accomplish the transformations of the unit-cell; in particular, blue arrows indindicate the portion that delivers the homogeneous shear.eTwin embryo structure generated by the P → B transformation, which shows a minor rotational deviation compared with the ideal twinf. Angle of the minor rotation can be described by tan−1(s/2), wheresis the magnitude of twinning shear (see Supplementary Fig.2for the derivation). 5 . e Mapping of the strain normal to the parent prismatic plane ( ε yy ) generated by the dislocation core, by geometrical phase analysis. Boxed region is the reference region for the geometrical phase analysis (see ref. [56] for more details). f – g Inverse fast Fourier transformations of the TEM snapshots in b , c , respectively, using the (0 0 0 1) reflections of the twin (indicated by turquoise-circles in h ). Turquoise dotted circles in b , c , f , g mark the twin embryo. White circles and lines in h indicate the reciprocal lattice of the matrix. Scale bars in a – d , 2 nm. 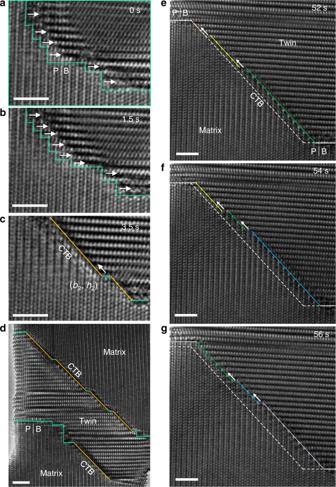Fig. 4: Twin boundary transformation from P│B interfaces to CTB during detwinning. a–cSequential HRTEM snapshots of the process. The dominant defects in the twinning transit from disconnections on P│B interfaces to twinning dislocations (b2,h2) on CTB. Zig-zag turquoise lines indicate the P│B interfaces. White arrows ina,bindicate the moving directions of the disconnections on the P│B interface.dOverview of the twin upon partial detwinning, showing serrated twin boundaries.e–gSequential HRTEM snapshots showing CTB propagation by twinning dislocations. White dash line is a reference line to show the migration of the CTBs (colored lines). Arrows inc,e–gindicate the migration direction of the twinning dislocations. Scale bars ina–g, 2 nm. 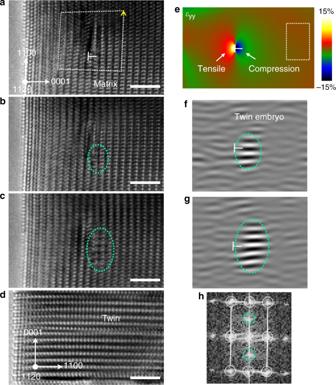Fig. 5: Twinning nucleation assisted by the strain field of a matrix dislocation. a–dSequential HRTEM images showing the nucleation of a twin embryo near the dislocation core (indicated by the “├” symbol). The crystal was under <1 −1 0 0 > -oriented compression and viewed along the <1 1 −2 0> direction. White dashed line inais the Burgers circuit which indicates an <a> component in the Burgers vector (indicated by the yellow arrow) of the dislocation. Detailed analysis of the Burgers vector is shown in Supplementary Fig.5.eMapping of the strain normal to the parent prismatic plane (εyy) generated by the dislocation core, by geometrical phase analysis. Boxed region is the reference region for the geometrical phase analysis (see ref.56for more details).f–gInverse fast Fourier transformations of the TEM snapshots inb,c, respectively, using the (0 0 0 1) reflections of the twin (indicated by turquoise-circles inh). Turquoise dotted circles inb,c,f,gmark the twin embryo. White circles and lines inhindicate the reciprocal lattice of the matrix. Scale bars ina–d, 2 nm. Full size image Through direct atomic scale observation, we discovered that nucleation of the predominant {1 0 −1 2} twinning is completed in two steps: I. Establishing the lattice correspondence through an interfacial process that directly transforms the parent prismatic plane into a twin basal plane; II. Correction of residual misorientation through rearrangement of the interfacial defects and ensuing formation of CTBs. In addition, the role of matrix dislocations on the twinning nucleation and direct evidence to the operation of the classical twinning dislocations are also revealed. The mechanism is expected to be present in bulk HCP metals, providing a solid fundamental basis for the twinning-based design and processing of HCP alloys. Fundamentally, this mechanism suggests that nucleation of twinning (or martensitic transformation) is essentially a transformation process that conforms to and establishes the lattice correspondence, which can be accomplished by many interfacial processes other than the classical twinning dislocations on the twinning (or habit) plane. In situ TEM experimental procedures Rhenium is widely used in structure materials in jet engines [58] , with outstanding mechanical properties and excellent oxidation resistances at high temperatures. Moreover, Re is resistant to electron irradiation [59] , making it a suitable model material for in situ TEM investigations. Re rods with 99.999% purity (ESPI metals) were cut into nanosized tips and loaded onto both the fixed-end and the piezo-end of a Nanofactory holder. Then, the nanotips were manipulated to touch each other inside the high vacuum (~10 −8 mbar) of a TEM and welded together by using an electric pulse. Then, the crystals were deformed by straining at a controlled rate of 10 −3 ~10 −4 /s. FEI 80-300 Titan equipped with a imaging lens spherical aberration corrector was used throughout this work. A charge-coupled device was used to record the images and videos (at two frames per second).